SNARE-fusion mediated insertion of membrane proteins into native and artificial membranes Membrane proteins carry out functions such as nutrient uptake, ATP synthesis or transmembrane signal transduction. An increasing number of reports indicate that cellular processes are underpinned by regulated interactions between these proteins. Consequently, functional studies of these networks at a molecular level require co-reconstitution of the interacting components. Here, we report a SNARE protein-based method for incorporation of multiple membrane proteins into artificial membrane vesicles of well-defined composition, and for delivery of large water-soluble substrates into these vesicles. The approach is used for in vitro reconstruction of a fully functional bacterial respiratory chain from purified components. Furthermore, the method is used for functional incorporation of the entire F 1 F 0 ATP synthase complex into native bacterial membranes from which this component had been genetically removed. The novel methodology offers a tool to investigate complex interaction networks between membrane-bound proteins at a molecular level, which is expected to generate functional insights into key cellular functions. Membrane proteins (MPs) are involved in a wide range of cellular processes such as molecular communication, sensation, transport and energy conversion, making them a major drug target [1] . Consequently, the molecular understanding of this class of proteins is of wide interest within both basic and applied sciences. In the past two decades, increasing numbers of crystal structures of MPs have been solved, which greatly improved our understanding of the structural and functional properties of MPs. However, crystal structures of MPs are typically obtained in detergents in the enzyme’s resting state and do not show the enzyme at work. It is thus essential to complement MP structures with functional studies, where the MP is at work preferably in a membrane that mimics the natural environment. Consequently, a common approach involves MP reconstitution in artificial bilayers such as liposomes, which mimic the cellular milieu and organization, that is, two compartments separated by a protein-containing lipid bilayer [2] , [3] . However, cellular functions are often underpinned by complex interactions between multiple membrane proteins, which requires co-reconstitution of multiple proteins. This approach presents a great challenge because reconstitution of purified MPs into lipid bilayers has to be optimized for every single protein. Not surprisingly, only very few examples of in vitro functional membrane protein co-reconstitutions are described [4] , [5] , [6] , [7] , [8] . Furthermore, some MPs interact functionally with water-soluble partners that must be delivered to the inside of vesicles after reconstitution, which is typically not possible. An example of a functional interplay of multiple MPs is exhibited by the members of the respiratory chain (complexes I–IV) and the ATP synthase (complex V) in mitochondria and aerobic bacteria that results in the production of ATP [9] . The respiratory chain enzymes use electrons delivered by NADH or succinate to reduce molecular oxygen to water, and exploit the free energy of this exergonic reaction to maintain a proton motive force (pmf) that drives the rotary mechanism of the ATP synthase [10] . Except for the co-reconstitution of the light-driven proton pump bacteriorhodopsin and ATP synthase [2] , [4] , in vitro studies investigating the interplay between the different members of the energy conversion machinery are lacking, mainly because of the difficulties described above. Here, we use MPs of bacterial respiratory chains as a model system to develop a novel methodology used to co-reconstitute multiple MPs. The general approach is based on the use of purified SNARE proteins, to deliver liposome-reconstituted MPs to artificial and native membrane fractions. The principle is to reconstitute each protein separately in liposomes (here, the protocol can be optimized for the particular protein, for example, with respect to orientation within the membrane or activity) and then fuse the different MP-containing vesicles to build a vesicle containing multiple MPs with unaltered orientation of each of the components. The liposomal fusion is mediated by so called v- and t-SNARE proteins (vesicle- and target-SNARE protein, respectively) that are added during or after the reconstitution of the desired MP into the liposomes. The v- and t-SNARE proteins are part of the fusion machinery in synaptic vesicles and have been found to be sufficient for mediating membrane fusion in vitro . The fusion process is presumably driven by the free energy of a four-helix bundle formation on v- and t-SNARE interaction [11] , [12] . The method is validated by demonstration of the successful co-reconstitution of three integral MPs, respiratory complexes II, IV and V, capable of ATP synthesis driven by succinate oxidation and oxygen reduction. We further apply the same technology to deliver the 15 kDa water-soluble protein cytochrome c (cyt. c ) into preformed proteoliposomes. Finally, ATP synthase reconstituted in vesicles is embedded functionally into native inverted membranes of an E. coli strain lacking ATP synthase, restoring respiratory-driven ATP synthesis. The described experiments comprise progress towards a step-by-step assembly of complex liposomal mixtures, including the possibility to deliver intact MPs into native membranes. Reconstitution of a single protein in liposomes In order to reconstitute MPs in liposomes, preformed lipid vesicles were mixed with the ionic detergent sodium cholate and the MP, triggering the formation of a ternary complex consisting of vesicles, detergent and enzyme [2] . After incubation, the detergent was removed by gel filtration or dialysis, yielding a bilayer-embedded MP. Other methods described for SNARE reconstitution including usage of Triton X-100 and Bio-Beads or freeze-thaw procedures are also likely to work [3] , [13] , but have not been investigated here. For both ATP synthase and bo 3 oxidase, we found that typically ~50% of the added proteins were reconstituted ( Supplementary Fig. 1 ). Co-reconstitution of two MPs by fusion In a first set of experiments, we reconstituted purified E. coli ubiquinol bo 3 oxidase, together with the v-SNARE synaptobrevin in one set of vesicles, and the E. coli ATP synthase together with the t-SNARE SNAP-25/syntaxin in another set of vesicles. The two populations were then mixed to initiate fusion ( Fig. 1a ). After ~20 min, turnover of the bo 3 oxidase was initiated on addition of the electron donors DTT (dithiothreitol) and water-soluble ubiquinol Q 1 . This reaction resulted in establishment of a pmf across the membrane. Synthesis of ATP was monitored continuously in a luminometer using a luciferin/luciferase system ( Fig. 1b ). The light intensity increased linearly with time, which implies that ATP was formed continuously. This increase was impaired on addition of potassium cyanide (KCN) or HQNO (2-heptyl-4-hydroxy quinoline-N-oxide), which block the catalytic site or interfere with ubiquinol binding, respectively, in the bo 3 oxidase ( Fig. 1b,c ). Because ATP synthesis driven by proton pumping by the bo 3 oxidase can only occur in the presence of a proton tight and intact bilayer, the data show that a complete vesicle fusion had occurred. Control experiments, in which one of the SNARE proteins was absent, showed no ATP production ( Fig. 1c ). Fusion was monitored over a time of ~60 min, showing consistency with earlier kinetic studies of SNARE-mediated fusion ( Fig. 1d ) [14] . 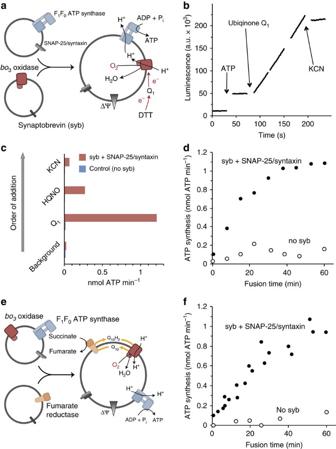Figure 1: SNARE-mediated reconstitution of multiple MPs. (a) Cartoon illustrating the experimental setup. The two liposomes populations were allowed to fuse for 20 min andbo3oxidase turnover was started with the addition of DTT/Q1. (b) Raw data obtained from luminometer measurements described in a. Indicated are the additions during the experiment. (c) ATP synthesis rates measured after different additions as indicated in b (red). Controls without synaptobrevin are also shown (blue). (d) Time course of fusion during the experiment described in a. ATP synthesis rates were determined at the indicated time points in the presence (closed circles) or absence of synaptobrevin (open circles). The experiment was repeated more than five times with different liposome and protein preparations. Essentially identical results were obtained. Shown are data from a single, typical experiment. (e) Reconstitution of an intact bacterial respiratory chain. After fusion, the experiment was initiated by addition of succinate, the substrate of complex II, reducing ubiquinone Q10and thus energizingbo3oxidase. (f) Time course of the experiment described in e. ATP synthesis rates were determined at the indicated time points in the presence (closed circles) or absence (open circles) of synaptobrevin. The experiment was performed twice with different liposome preparations. Essentially identical results were obtained. Data from two experiments with the same liposome preparation are shown. Figure 1: SNARE-mediated reconstitution of multiple MPs. ( a ) Cartoon illustrating the experimental setup. The two liposomes populations were allowed to fuse for 20 min and bo 3 oxidase turnover was started with the addition of DTT/Q 1 . ( b ) Raw data obtained from luminometer measurements described in a. Indicated are the additions during the experiment. ( c ) ATP synthesis rates measured after different additions as indicated in b (red). Controls without synaptobrevin are also shown (blue). ( d ) Time course of fusion during the experiment described in a. ATP synthesis rates were determined at the indicated time points in the presence (closed circles) or absence of synaptobrevin (open circles). The experiment was repeated more than five times with different liposome and protein preparations. Essentially identical results were obtained. Shown are data from a single, typical experiment. ( e ) Reconstitution of an intact bacterial respiratory chain. After fusion, the experiment was initiated by addition of succinate, the substrate of complex II, reducing ubiquinone Q 10 and thus energizing bo 3 oxidase. ( f ) Time course of the experiment described in e. ATP synthesis rates were determined at the indicated time points in the presence (closed circles) or absence (open circles) of synaptobrevin. The experiment was performed twice with different liposome preparations. Essentially identical results were obtained. Data from two experiments with the same liposome preparation are shown. Full size image In similar experiments, we varied the number of SNARE proteins (while keeping a 1:1 ratio of synaptobrevin and SNAP-25/synthaxin) and followed ATP synthesis driven by the bo 3 oxidase (as outlined above). The optimal number of SNARE proteins per vesicle was found to be in the range of 10–50 ( Supplementary Fig. 2 ). In addition, liposomes of different size (diameters in the range 30–200 nm) were successfully tested (data not shown). Effect of lipid composition on fusion efficiency Soybean asolectin is a commonly used lipid source for membrane protein reconstitution and was used in the experiment above. However, its detailed composition is undefined and because the extract is relatively crude, other molecules than lipids (for example, fusogenic agents) may be present. We thus tested the efficiency of SNARE-mediated liposome fusion also with other lipid compositions such as extracts from the E. coli membrane and a variety of synthetic lipid combinations. One such mixture contained 40% dioleoyl-phosphatidyl choline (DOPC), 20% dioleoyl-phosphatidyl ethanolamine, 20% dioleoyl-phosphatidyl glycerol, 10% sphingomyelin, 10% cholesterol, approximately imitating the lipid composition of a eukaryotic plasma membrane. Furthermore, we reconstituted ATP synthase and SNAP-25/synthaxin in liposomes made from 100% DOPC and mixed them with bo 3 oxidase and synaptobrevin-containing liposomes composed of different lipids as indicated in Fig. 2 . Successful fusion was observed in all tested cases, indicating that the process is essentially independent of lipid composition. It is not clear from our experiments, however, if the observed differences (60–120% ATP synthesis activity compared to that obtained with DOPC:DOPC fusion) are a consequence of different fusion efficiencies or a direct lipid dependence on the coupled activity of the bo 3 oxidase and the ATP synthase (for example, proton coupling). With lipids from natural sources, slightly higher activities were obtained ( Fig. 2 , dark grey bars). As all lipids were weighed in dried form, the phospholipid content (per mg powder) from natural sources is expected to be lower than from synthetic lipids. This can result in a different number of liposomes and thus influence the protein per liposome ratio. Less activity was found in the negative control with synthetic lipids (DOPC:DOPC, no synaptobrevin) compared with natural lipids (soybean:DOPC, no synaptobrevin). This observation might indicate that soybean asolectin indeed contains a small amount of a fusogenic agent, mediating liposome fusion in the absence of synaptobrevin. 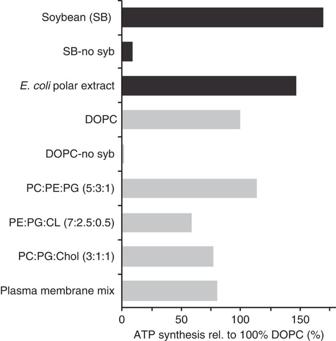Figure 2: Effect of lipid composition on SNARE-mediated fusion. Shown are the relative ATP synthesis rates after fusion of ATP synthase in 100% DOPC liposomes withbo3liposomes composed of different lipid compositions (the rate with 100% DOPC is set as 100%). Slightly different liposome concentrations are possible from dried natural lipid extracts (dark grey) and mixtures of synthetic lipids (light grey). Control experiments without SNARE protein synaptobrevin are indicated (no syb). The experiment has been performed twice with different liposome preparations. Essentially identical results were obtained. Shown are averaged data from two measurements with one liposome preparation. Figure 2: Effect of lipid composition on SNARE-mediated fusion. Shown are the relative ATP synthesis rates after fusion of ATP synthase in 100% DOPC liposomes with bo 3 liposomes composed of different lipid compositions (the rate with 100% DOPC is set as 100%). Slightly different liposome concentrations are possible from dried natural lipid extracts (dark grey) and mixtures of synthetic lipids (light grey). Control experiments without SNARE protein synaptobrevin are indicated (no syb). The experiment has been performed twice with different liposome preparations. Essentially identical results were obtained. Shown are averaged data from two measurements with one liposome preparation. Full size image Functional co-reconstitution of three MPs In the next experiment, the artificial, water-soluble electron donor ubiquinone Q 1 was replaced with a native lipid-soluble analogue, ubiquinone Q 10 ( E. coli uses Q 8 ). Under physiological conditions (in an aqueous solvent), long-chain ubiquinones such as Q 10 can only be enzymatically reduced, for example, in E. coli by complex I (NADH:Q oxidoreductase) or one of the two variants of complex II (succinate:formate dehydrogenase or fumarate reductase [15] ). The latter was purified and reconstituted in vesicles containing 1% (w/w) ubiquinol Q 10 and v-SNARE synaptobrevin. In another sample, ATP synthase and bo 3 oxidase were co-reconstituted in vesicles containing 1% (w/w) ubiquinol Q 10 and t-SNARE SNAP-25/syntaxin. The two liposome samples were mixed and allowed to fuse before succinate, the substrate of complex II, was added ( Fig. 1e ). Because the reaction catalysed by complex II is not electrogenic, formation of a pmf across the membrane can only occur on turnover of the bo 3 oxidase, which is driven by ubiquinol Q 10 that has to be reduced by complex II. As seen in Fig. 1f , ATP synthesis was indeed observed, demonstrating that all three enzymes are present in the same membrane. The increase in the ATP-driven light intensity occurred over the same time range as for the two-component system described above ( cf . Fig. 1d ). However, the ATP synthesis rates were slower than in the experiments with only two enzymes, presumably because the overall turnover rate is determined by that of complex II, which is only ~30 e − s −1 with ubiquinone Q 1 as an electron acceptor [16] (in contrast to >300 e − s −1 with Q 1 /DTT for the bo 3 oxidase [17] ). Again, essentially no ATP synthesis activity was observed in the absence of synaptobrevin ( Fig. 1f ) or in the absence of Q 10 in the liposome. In the latter case, a residual activity of <15% was observed, which is likely to be explained by natural quinones present in the soybean lipid preparation. Delivery of a 15 kDa protein into intact proteoliposomes We further exploited the potential of SNARE-controlled liposome fusion for delivery of membrane-impermeable proteins into intact vesicles. In mitochondria and in many bacteria, a cytochrome c oxidase (Cyt c O) is used instead of a quinol oxidase as the terminal electron acceptor. The use of a Cyt c O in a coupled in vitro system with the ATP synthase is, however, accompanied by a complication. It has been found that on reconstitution in vesicles, ATP synthase is exclusively oriented with the headpiece towards the outside [18] and, therefore, protons have to be pumped into the vesicles to create the pmf required for ATP synthesis. Consequently, only Cyt c Os with the cyt. c binding domain on the inside of the liposomes contribute to maintain the correct gradient, which requires that reduced cyt. c has to be available inside of the liposomes. To test whether the above-described fusion method could be used to deliver cyt. c into liposomes, we prepared one sample with vesicles containing ~20 μM cyt. c inside the vesicles and synaptobrevin in the membrane. This sample was mixed with vesicles containing membrane-reconstituted Cyt c O ( aa 3 -type) from R. sphaeroides , ATP synthase from E. coli and SNAP-25/syntaxin ( Fig. 3a ). Reduction of the vesicle-encapsulated cyt. c 3+ was achieved by addition of ascorbate and the membrane-permeable electron mediator phenazine methosulfate (PMS) to the outside of the vesicles. Because the ascorbate/PMS mixture also slowly reduces Cyt c O directly, the ATP-formation rates were compared with those obtained after fusion with empty vesicles (with synaptobrevin in the membrane). ATP synthesis was about a factor of five faster in the presence of cyt. c compared to ascorbate/PMS only ( Fig. 3b ), demonstrating successful delivery of cyt. c to the target vesicles. 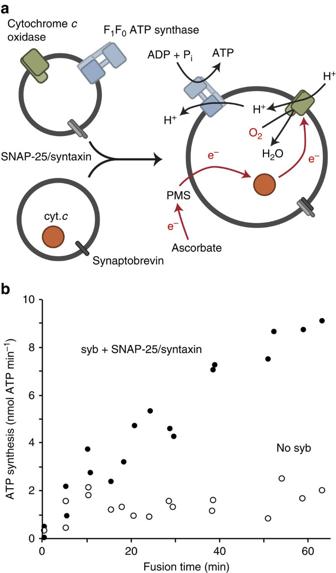Figure 3: Delivery of cyt.cinto liposomes containing CytcO and ATP synthase. (a) Cartoon illustrating the experimental setup. Liposomes containing soluble cyt.cand synaptobrevin were mixed with proteoliposomes containing CytcO oxidase, ATP synthase and SNAP-25/syntaxin. The reaction was started by the addition of ascorbate and PMS as electron donor and mediator, respectively. (b) Time course displaying the stimulated ATP synthesis activity after fusion of the two liposome populations in the presence (filled circles) and absence (open circles) of synaptobrevin. The low, but constant activity found in the sample without synaptobrevin is due to direct reduction ofbo3oxidase by ascorbate/PMS. The experiment has been performed with three different liposome preparations. Shown are the combined data from two measurements of the same liposome preparation. Figure 3: Delivery of cyt. c into liposomes containing Cyt c O and ATP synthase. ( a ) Cartoon illustrating the experimental setup. Liposomes containing soluble cyt. c and synaptobrevin were mixed with proteoliposomes containing Cyt c O oxidase, ATP synthase and SNAP-25/syntaxin. The reaction was started by the addition of ascorbate and PMS as electron donor and mediator, respectively. ( b ) Time course displaying the stimulated ATP synthesis activity after fusion of the two liposome populations in the presence (filled circles) and absence (open circles) of synaptobrevin. The low, but constant activity found in the sample without synaptobrevin is due to direct reduction of bo 3 oxidase by ascorbate/PMS. The experiment has been performed with three different liposome preparations. Shown are the combined data from two measurements of the same liposome preparation. Full size image Absolute yield of SNARE-mediated fusion Using a similar setup as in Fig. 3 , we quantified the yield of vesicle fusion. Reports on fusion yields of empty vesicles are rare, as typically only qualitative results are presented, but electron microscopy or fluorescence microscopy have been applied and high fusion efficiencies of up to 80% have been reported [19] , [20] . In our experiment, we entrapped pre-reduced cyt. c in vesicles containing synaptobrevin and removed the non-entrapped cyt. c by means of a cation exchange column. These vesicles were then fused with another set of vesicles containing Cyt c O and SNAP-25/syntaxin. Electron transfer from cyt. c to Cyt c O would only occur after interaction of the cyt. c binding domain of Cyt c O with cyt. c and thus only after successful fusion. The reduction state of cyt. c was monitored spectrophotometrically at 550 nm. As depicted in the inset of Fig. 4 , a decrease in absorbance at 550 nm was observed on mixing of the two liposome populations. The absorbance decrease displayed similar kinetics to that observed for vesicle fusion in all our experiments. After 120 min, membrane-impermeable ferricyanide (Fe 3+ ) was added and no further decrease was observed, indicating that no external cyt. c was present. On addition of the membrane-permeable electron mediator PMS, the remaining part of cyt. c was oxidized by the ferricyanide. The data indicate fusion yields of ~70%. This number is likely an underestimate as, for example, complete oxidation of cyt. c is unlikely in the absence of a strong electron sink such as ferricyanide. Furthermore, it is likely that some fusion events do not generate a signal because of lack of correctly oriented Cyt c O. 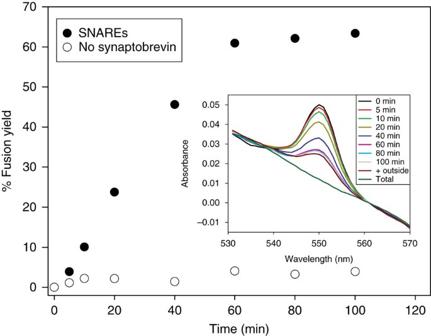Figure 4: Estimate of the fusion yield. Absorbance changes were measured during fusion of vesicles containing synaptobrevin and entrappedcyt. c, and vesicles containing CytcO. Time course of absorbance changes at 550 nm, recalculated into the fusion yield as outlined in the text. Shown is the kinetics for liposomes containing 20 SNAREs per liposome (full circles) and liposomes containing no synaptobrevin (open circles). Original absorption spectra (inset) after different time points and after addition of the membrane-impermeable electron acceptor ferricyanide (+outside) and the membrane-permeable electron mediator PMS (total). The experiment has been performed twice with two different liposome preparations with very similar results. Data from one experiment are shown. Figure 4: Estimate of the fusion yield. Absorbance changes were measured during fusion of vesicles containing synaptobrevin and entrapped cyt. c , and vesicles containing Cyt c O. Time course of absorbance changes at 550 nm, recalculated into the fusion yield as outlined in the text. Shown is the kinetics for liposomes containing 20 SNAREs per liposome (full circles) and liposomes containing no synaptobrevin (open circles). Original absorption spectra (inset) after different time points and after addition of the membrane-impermeable electron acceptor ferricyanide (+outside) and the membrane-permeable electron mediator PMS (total). The experiment has been performed twice with two different liposome preparations with very similar results. Data from one experiment are shown. Full size image Incorporation of purified synaptobrevin in intact bilayers In all the above-described experiments, SNARE proteins were introduced together with the desired MP reconstitution into liposomes. However, it might be advantageous to incorporate SNARE proteins into already existing bilayer structures (giant liposomes, planar bilayers or native membrane vesicles). We therefore tested whether or not the smaller SNARE protein synaptobrevin (~18 kDa, one transmembrane helix) inserts spontaneously into membranes when added to preformed liposomes. While liposomes containing ATP synthase and SNAP-25/syntaxin were prepared as described for the experiments shown in Fig. 1 , synaptobrevin was either added during or after reconstitution of bo 3 oxidase into liposomes. Spontaneous incorporation of synaptobrevin was then monitored via ATP synthesis activity as a result of successful fusion of the two populations. No detectable ATP synthesis was observed after 30 min of fusion, when 10 synaptobrevin molecules per vesicles were added after reconstitution (data not shown). Only when the synaptobrevin amount was raised fivefold, 25% of the activity of the co-reconstituted sample was found ( Fig. 5 , c.f. columns B and D). While sonication of the bo 3 liposomes/synaptobrevin mixture did increase activity only marginally ( Fig. 5 , column E), the presence of a low concentration (0.05%) of the ionic detergent Na-cholate greatly enhanced the incorporation efficiency (110% of the control activity, Fig. 5 , column F). No further activation was observed, when the cholate-supplied sample was sonicated ( Fig. 5 , column G). Essentially no activity was observed when synaptobrevin was omitted, in the absence ( Fig. 5 , column A) or presence of cholate ( Fig. 5 , column C). 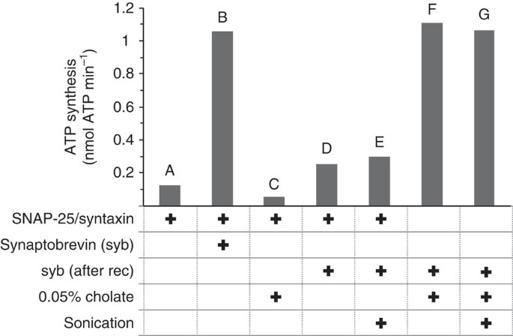Figure 5: Post-reconstitution insertion of synaptobrevin into liposomal membranes. Shown are the ATP synthesis activities of different reconstitution conditions. The liposome and membrane protein concentration were constant. Shown are the averaged results from two experiments with different liposome preparations. Figure 5: Post-reconstitution insertion of synaptobrevin into liposomal membranes. Shown are the ATP synthesis activities of different reconstitution conditions. The liposome and membrane protein concentration were constant. Shown are the averaged results from two experiments with different liposome preparations. Full size image Functional insertion of ATP synthase into E. coli membranes Motivated by the finding that the small SNARE protein synaptobrevin can be incorporated into a pre-existing membrane without affecting bilayer integrity, we aimed to translate this methodology to native bacterial membranes ( Fig. 6a ). For this study, E. coli strains BL21 and DK8 were grown, where the latter lacks the complete atp operon and thus the ATP synthase. Inverted membrane vesicles were prepared that can be used to measure ATP synthesis either on addition of NADH (to initiate electron transfer from complex I) [21] or DTT/Q 1 (to initiate electron transfer from bo 3 oxidase) [22] . As expected, both strains exhibited respiratory enzyme activity ( Fig. 6b , inset), but only strain BL21 showed ATP synthesis on addition of the electron donors (not shown). We found ATP synthesis rates of ~0.2 and ~0.7 μmol ATP mg −1 protein min −1 when inverted membrane vesicles were energized with NADH and Q 1 /DTT, respectively. The former value is in very good agreement with that obtained in the study of Etzold et al . [21] assuming an ATP synthase content of 5% of the total membrane protein. Interestingly, when respiration was driven with Q 1 /DTT, a fourfold higher ATP synthase activity was found, corroborating the finding of Etzold et al . [21] that ATP synthesis is underpowered when driven with NADH alone. Analogously to the experiments described above, the DK8 membrane fraction (lacking ATP synthase) was doped with synaptobrevin in the presence of 0.05% Na-cholate. When mixed with liposomes containing ATP synthase and SNAP-25/syntaxin, the DK8 membranes showed SNARE-dependent ATP synthesis on addition of NADH or DTT/Q 1 (up to 40% of that observed with strain BL21), demonstrating the incorporation of fully functional ATP synthase into E. coli inverted vesicles ( Fig. 6b ). A prerequisite for this experiment was to insert synaptobrevin into the native membrane, which was achieved by a mild treatment of the membrane with a low concentration of Na-cholate (0.05%), a detergent with a very high critical micellar concentration (~0.8%). Consequently, the integrity of the membrane was not affected. An extension of this methodology could involve genetic expression of synaptobrevin (or another SNARE molecule) in the target vesicle. 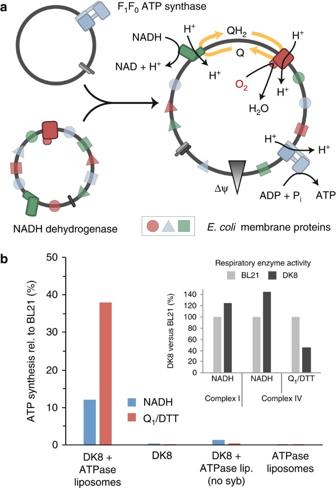Figure 6: Insertion of ATP synthase into inverted membrane vesicles ofE. coli. (a) Cartoon illustrating the experimental setup. Inverted membrane vesicles ofE. coliDK8 doped with synaptobrevin were mixed with liposomes containing ATP synthase and SNAP-25/syntaxin and allowed to fuse. (b) Respiratory-driven ATP synthesis after fusion as described in a. The results are given compared with a similar preparation of strain BL21, normalized to the total membrane protein concentration. Hundred percent ATP synthesis activity in wt BL21 membranes corresponds to 4.6 nmol ATP min−1and 20.4 nmol ATP min−1when energized with complex I andbo3oxidase, respectively. Shown are the relative activities after addition of NADH (blue) and DTT/Q1(red). Relative respiratory enzyme activities in inverted membranes of strains BL21 (light grey) and DK8 (dark grey) measured as NADH oxidation for complex I and O2consumption for complex IV (driven by either NADH oxidation or DTT/Q1) are also shown (inset). The experiment has been performed three times with different membrane and liposome preparations with very similar results. Shown are the results from one experiment. Figure 6: Insertion of ATP synthase into inverted membrane vesicles of E. coli . ( a ) Cartoon illustrating the experimental setup. Inverted membrane vesicles of E. coli DK8 doped with synaptobrevin were mixed with liposomes containing ATP synthase and SNAP-25/syntaxin and allowed to fuse. ( b ) Respiratory-driven ATP synthesis after fusion as described in a. The results are given compared with a similar preparation of strain BL21, normalized to the total membrane protein concentration. Hundred percent ATP synthesis activity in wt BL21 membranes corresponds to 4.6 nmol ATP min −1 and 20.4 nmol ATP min −1 when energized with complex I and bo 3 oxidase, respectively. Shown are the relative activities after addition of NADH (blue) and DTT/Q 1 (red). Relative respiratory enzyme activities in inverted membranes of strains BL21 (light grey) and DK8 (dark grey) measured as NADH oxidation for complex I and O 2 consumption for complex IV (driven by either NADH oxidation or DTT/Q 1 ) are also shown (inset). The experiment has been performed three times with different membrane and liposome preparations with very similar results. Shown are the results from one experiment. Full size image The results from this study show that SNARE proteins can be used as a tool to insert MPs in the lipid bilayer of artificial and native membranes in a controlled manner. To our knowledge, this is not only the first study describing a complete in vitro reconstituted respiratory chain, but also the first co-reconstitution of three multisubunit MPs in the same vesicular membrane. Furthermore, we successfully demonstrate the functional insertion of a fully folded multisubunit protein into the densely packed native bilayer of inverted E. coli membranes. The method further allows delivery of relatively large water-soluble components (in this case the 15 kDa protein cyt. c ) across an intact bilayers into, for example, a liposome. Under the described conditions, fusion yields of ~70% with a variety of lipid sources were achieved, reinforcing the broad applicability of the method. The stalk hypothesis for SNARE-mediated fusion predicts that fusion occurs in three steps. First, v- and t-SNARE proteins interact and bring the two membranes in close proximity before fusion of the outer membrane leaflets starts. The process might halt temporarily in a state called hemi-fusion, where no content exchange of the two compartments is possible. Finally, pore opening starts and the two membranes fuse completely to reform one larger vesicle [12] . Because ATP synthesis requires the presence of an electrochemical proton gradient, our data demonstrate that complete fusion occurs and a continuous intact membrane bilayer is formed. The fusion model described above also predicts that the MPs maintain their orientation on fusion. This is corroborated by the successful co-reconstitution of ATP synthase that has been shown to insert unidirectionally with the F 1 head part on the outside of liposomes [18] . Consequently, the reconstitution protocol can be optimized for a specific orientation for each membrane protein separately rather than for all the co-reconstituted proteins at the same time. The presence of either v- or t-SNAREs in each liposome population ensures that only the desired combination of MPs occurs. Unfortunately, for most MPs (for example, bo 3 oxidase, Cyt c O), unidirectional incorporation is not readily controlled, but ongoing work is aimed at developing protocols for unidirectional orientation, as a homogenous distribution of enzymes in the proteoliposomes is a prerequisite for a determination of the coupling efficiency between the co-reconstituted enzymes. While synaptobrevin and SNAP-25/syntaxin is the best-characterized SNARE couple, also other SNAREs have been described and studied [12] . Thus, an extension of the approach described may be to use a combination of different SNARE couples for multiple, consecutive fusion processes. The method also allowed us to successfully incorporate a fully folded multisubunit membrane protein into an existing native membrane, densely packed with endogenous MPs. Thus, the same approach could also be used for in vitro introduction of new lipid components or labelled lipids into native membranes, which would make it possible, for example, to investigate dynamic aspects of specific protein–lipid interactions within the native membrane. Finally, the method nicely bridges in vitro characterization of specific MPs with in vivo studies of their roles in the native membrane. In the past years, several in vitro techniques have been described to initiate targeted membrane fusion [23] , including DNA-based techniques, where hybridization of complementary DNA strands is used to bring membranes into close proximity [24] , [25] . The high variability of DNA sequences makes this a very promising approach for highly specific fusion processes. In comparison with SNARE-mediated fusion events, however, DNA-based assays showed leakage during the fusion process. No leakage was found in a further alternative using lipid-bound peptides (separated by a polyethylene glycol spacer) that form strong coiled coil structures mimicking the four-helix bundle of natural SNARE proteins [26] . Using different peptide sequences for specific recognition, these synthetically prepared lipid–peptide construct might be a valuable alternative to natural SNARE proteins. cyt. c and ubiquinol oxidases cyt. c oxidase from Rhodobacter sphaeroides was purified as previously described [27] . The bo 3 oxidase from E. coli was expressed from plasmid pETcyo expressed in strain C43 and purified as described [28] . Fumarate reductase from E. coli Fumarate reductase was purified from plasmid pH53, a derivative of pH3 including a 6xHis-Tag at the C-terminus of FrD, expressed in strain BW35 (ref. 29 ). Briefly, plasmid pH53 was transformed into strain BW35 using Ampicillin (200 μg ml −1 ) and Kanamycin (50 μg ml −1 ) as antibiotics. Expression was done in 4.5 l Terrific Broth containing Ampicillin (200 μg ml −1 ) at 37 °C, 120 r.p.m. (microaerobic conditions) overnight. Half of the cells (~7 g) were resuspended in a 60 ml buffer containing 50 mM Hepes, pH 7.5, 150 mM KCl, DNaseI and disrupted by French Press (2 × 10,000 psi). Cell debris was removed by low-spin centrifugation (8,000 g , 4 °C, 15 min) and the membranes were collected by ultracentrifugation (200,000 g , 4 °C, 90 min). Solubilization of the membranes (1 h, 4 °C) was performed in 15 ml buffer containing 20 mM Hepes, pH 7.5, 150 mM KCl, 1% Triton X-100. The supernatant after ultracentrifugation (150,000 g , 4 °C, 45 min) was mixed with 10 ml Ni-NTA column (50% slurry) and incubated on a slowly rotating wheel (1 h, 4 °C). The slurry was poured into an empty column and after sedimentation, the column was washed with 10 CV of buffer containing 20 mM Hepes, pH 7.5, 150 mM KCl, 0.1% Triton X-100 and with 10 CV of the same buffer containing 15 mM imidazole. The protein was eluted with buffer (the same buffer containing 50 mM imidazole), and the coloured fractions were pooled and concentrated. The protein was aliquoted, shock-frozen in LN 2 and stored at −80 °C. F 1 F 0 ATP synthase from Escherichia coli The protein was expressed from plasmid pBWU13-βHis in E. coli strain DK8 and purified as described [18] . Synaptobrevin and SNAP-25/Syntaxin complex Synaptobrevin and SNAP-25/Syntaxin complex were purified from Escherichia coli according to previously described protocols [30] , [31] . Liposome preparation Liposomes were prepared from soybean acolectin (Type II-S, Sigma). Lipids were resuspended to homogeneity in 20 mM HEPES, pH 7.5, 2.5 mM MgSO 4 , 50 g l −1 sucrose to a concentration of 10 mg ml −1 . For all experiments (see exception below), the liposomes were made by subjecting the lipid suspension to at least six freeze-thaw cycles followed by extrusion (~20 passages) through a 100-nm membrane. Liposomes used for fusion with membrane vesicles from E. coli were suspended from soybean asolectin, as described above. The lipid mixture was then sonicated in a probe sonicator (5 min total sonication, 30 s/30 s on/off-cycle). Lipid aggregates and titanium particles from the sonicator probe were removed by centrifugation (4,000 g , room temperature, 15 min). The diameter of the resulting liposomes was estimated to be ~40 nm. In the experiments involving ubiquinone Q 10 , it was added to asolectin lipids dissolved in chloroform. The chloroform was removed by evaporation (stream of N 2 , Speed-Vac, 2 h, no heating) and the liposomes were then formed according to the protocol described above. Liposome preparation from synthetic lipids The procedure for preparation of liposomes from synthetic lipids was essentially the same as that used with soybean asolectin, except that purified lipids (dissolved at 20 mg ml −1 in chloroform) were mixed in a 5-ml round bottomed flask and the chloroform was evaporated under a stream of nitrogen, while the flask was rotated to achieve an evenly distributed thin layer of lipids. The lipids were then further dried under vacuum for 2 h, before they were resuspended (lipids were allowed to hydrate for at least 30 min) at a concentration of 10 mg ml −1 in 20 mM HEPES, pH 7.5, 2.5 mM MgSO 4 , 50 g l −1 sucrose. Liposome concentration calculation The liposome concentration was estimated by division of the lipid concentration by the number of lipids needed to form one liposome. This was done by calculating the volume of the membrane of the liposome (assuming a membrane thickness of 6 nm) and dividing by the volume of a single lipid (DOPC, 1300.1 Å 3 ) [32] . The liposome concentration of the 100 nm and 40 nm liposomes in a 10 mg ml −1 lipid suspension were estimated to be 0.12 μM and 0.85 μM, respectively. Preparation of inverted membrane vesicles from E. coli Escherichia coli cells (strain BL21 or DK8 (lacking the atp operon)) were grown overnight in LB medium into stationary phase (37 °C, 180 r.p.m.) and collected by centrifugation (15 min, 4 °C) 8,000 g . The cells were resuspended in 100 mM HEPES pH 7.5, 5 mM MgSO 4 , 100 mM KCl and disrupted by passing through a French press (2 × 11,000 psi) in the presence of protease inhibitor phenylmethylsulfonyl fluoride and DNaseI, rendering inside-out membrane vesicles [33] . Cell debris and whole cells were removed by low-spin centrifugation (8,000 g , 4 °C, 20 min) and the membrane vesicles were washed twice in 10 mM HEPES, 5 mM MgSO 4 , 100 mM KCl by ultracentrifugation (150,000 g , 4 °C, 1 h). Enzyme reconstitution General method: membrane protein reconstitution and SNARE reconstitution was performed mixing the enzymes with preformed liposomes in the presence of 0.6% sodium cholate for 30 min at room temperature. The detergent was removed by gel filtration on a PD-10 column (GE Healthcare), pre-equilibrated with 20 mM HEPES pH 7.5, 2.5 mM MgSO 4 , 50 g l −1 sucrose. Unless specified otherwise, 100 nm proteoliposomes (0.11 μM liposome concentration) were formed by mixing preformed liposomes containing 0.6% Na-cholate with the desired membrane protein (0.11 μM F 1 F 0 ATP synthase, 0.58 μM bo 3 oxidase, cyt. c oxidase, 0.11 μM fumarate reductase) and 1.17 μM synaptobrevin or SNAP-25/syntaxin complex. The final detergent concentrations in the reconstitution mixture (except 0.6% Na-cholate) were the following: ATP synthase (<0.02% Octyl-β-D-glucopyranoside, <0.02% Na-deoxycholate); bo 3 oxidase (<0.002% n-dodecyl β-D-maltoside); aa 3 ((<0.002% n-dodecyl β- D -maltoside); fumarate reductase (<0.002% Triton X-100). In control experiments, where one of the components was missing the difference in volume was adjusted with buffer. Liposomes used in investigating the effect of SNARE concentration were made using the same protocol but with either 0, 0.56, 1.12, 2.25 or 5.6 μM of the respective SNARE proteins. Liposomes loaded with cyt. c were made by including 30 μM cyt. c during reconstitution. After gel filtration, non-incorporated cyt. c was removed by passing the suspension through a weak cation exchange column (carboxymethyl-sepharose) that binds cyt. c tightly. In experiments, where synaptobrevin was added after enzyme reconstitution, proteoliposomes containing MPs (F 1 F 0 ATP synthase, bo 3 oxidase) were formed as described above. Synaptobrevin (6 μM) was then added to the liposomes either in the presence or absence of 0.05% sodium cholate. The samples were mixed for 30 min on a shaking table. A subset of the samples was subjected to 30 s sonication in a bath sonicator once every 5 min. Finally, the samples were run on a PD-10 gel filtration column to remove residual detergent. Liposome fusion Fusion of liposomes was performed by mixing the two samples of interest with occasional gentle shaking. A small portion of the sample was either taken at a fixed time point or incrementally over a longer time course, and its ATP synthesis activity was measured. ATP synthesis ATP formation by F 1 F 0 ATP synthase was determined using the luciferase/luciferin system [34] . Luminescence proportional to ATP concentration was measured with a luminometer (Glomax, Promega). Briefly, 500 μl of measuring buffer containing 20 mM Tris-PO 4 , pH 7.5, 2.5 mM MgCl 2 , 2 μl 20 mM ADP, 10 μl CLS luciferase (Roche Diagnostics), supplied with 10 μl proteoliposomes was used to record background activity of the luciferase under measurement conditions. In measurements, where the quinol bo 3 oxidase was used, 2 μl 1 M DTT was also included from the start and the reaction was started by the addition of 1 μl 10 mM ubiquinone Q 1 . In experiments with Cyt c O, 2 μl of 0.6 M ascorbate was included from the start and the reaction was started by the addition of 1 μl 5 mM PMS. In experiments with fumarate reductase, the reaction was started by addition of 5 μl 1 M succinate. Reactions driven by NADH dehydrogenase were started by the addition of 10 μl 10 mM NADH. Inhibition experiments were done by addition of either 8 μl 1 mM HQNO or 4 μl 40 mM potassium cyanide. Absorption spectroscopy To monitor the fusion progress, 250 μl liposomes containing Cyt c O (~five enzymes per vesicle) and SNAP-25/syntaxin was mixed in a 500-μl cuvette (at room temperature) with liposomes containing 50 μM cyt. c either with or without synaptobrevin (external cyt. c was removed by a passage of the liposomes through a weak cation exchange matrix). At specific time points (see Fig. 4 ), an absorption spectrum (530–570 nm) was recorded. After 100 min, 1 mM ferricyanide was added to oxidize residual cyt. c on the outside (not detectable). Finally, 1 μM PMS was added to shuttle electrons from cyt. c on the inside of liposome to ferricyanide on the outside. Complex I activity measurements Oxidation of NADH by complex I was followed in a spectrophotometer monitoring the decrease in absorbance of NADH at 340 nm under the same buffer conditions as in the ATP synthase measurements, but without luciferase. NADH dehydrogenase activity was initiated by addition of NADH (200 μM). Quinol oxidase activity The bo 3 quinol oxidase activity was determined in an oxygraph (Oxytherm, Hansatech) using the same conditions as in the ATP synthesis measurements, but without luciferase. Quinol oxidase activity was initiated either by addition of DTT/Q 1 (4 mM/20 μM) or NADH (200 μM). How to cite this article: Nordlund G. et al . SNARE-fusion mediated insertion of membrane proteins into native and artificial membranes. Nat. Commun. 5:4303 doi: 10.1038/ncomms5303 (2014).